3,3-Difluoroallyl ammonium salts: highly versatile, stable and selectivegem-difluoroallylation reagents 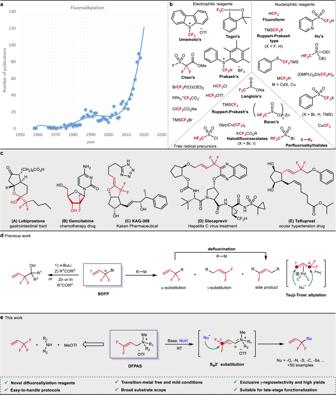Fig. 1: The allure of fluoroalkylations. aThe dynamic development of fluoroalkylations in the past years.bCommonly used fluoroalkyl-containing reagents for direct preparation of fluoroalkyl compounds.cThe importance of compounds containing difluoromethylene unit.dThe challenge of the direct preparation ofgem-difluoroallyl compounds using BDFP.eThe presented strategy for the selective construction ofgem-difluoroallyl compounds. The selective synthesis of fluorinated organic molecules continues to be of major importance for the development of bioactive compounds (agrochemicals and pharmaceuticals) as well as unique materials. Among the established synthetic toolbox for incorporation of fluorine-containing units, efficient and general reagents for introducing -CF 2 - groups have been largely neglected. Here, we present the synthesis of 3,3-difluoropropen-1-yl ammonium salts (DFPAs) as stable, and scalable gem -difluoromethylation reagents, which allow for the direct reaction with a wide range of fascinating nucleophiles. DFPAs smoothly react with N -, O -, S -, Se -, and C -nucleophiles under mild conditions without necessity of metal catalysts with exclusive regioselectivity. In this way, the presented reagents also permit the straightforward preparation of many analogues of existing pharmaceuticals. In general, the substitution of C–H bonds by C–F bonds in organic compounds leads to significant changes in their physical, chemical, and biological behavior. More specifically, properties such as solubility, metabolic stability, hydrogen-bonding ability, lipophilicity, and chemical reactivity are strongly influenced by the incorporation of fluorine atoms [1] , [2] , [3] , [4] . Hence, an increasing number of products of the pharmaceutical and agrochemical industries as well as material sciences [5] contain fluorine atoms as a crucial part [6] . Indeed, nearly 20% of the top 200 drugs in 2016 belong to this class of compounds [7] . Due to the dynamic development in this area more than 40% (45% and 41%) of FDA-approved drugs in 2018 [8] , and 2019 [9] are fluorine-containing. Even more pronounced, nearly 60% of the active ingredients for the agrochemical industry are fluorinated compounds. Not surprisingly, the incorporation of fluorine-containing groups has become one of the most important synthetic strategies for the design of new drugs and agrochemicals. Consequently, enormous efforts took place in academia and industry to develop such transformations [10] (Fig. 1a ), and many prominent fluoroalkylating agents containing CF 3 or related groups were successfully introduced in the past years [11] , [12] , [13] , [14] , [15] . A selection of privileged reagents is shown in Fig. 1b . Fig. 1: The allure of fluoroalkylations. a The dynamic development of fluoroalkylations in the past years. b Commonly used fluoroalkyl-containing reagents for direct preparation of fluoroalkyl compounds. c The importance of compounds containing difluoromethylene unit. d The challenge of the direct preparation of gem -difluoroallyl compounds using BDFP. e The presented strategy for the selective construction of gem -difluoroallyl compounds. Full size image In contrast to –CH 2 F or –CF 3 substituents, –CF 2 –R containing bioactive compounds are significantly less explored and comparably few marketed therapeutic agents exist yet (for some examples see Fig. 1c ) [16] , [17] , [18] , [19] , [20] , [21] , [22] , [23] . So far, the most common route for their synthesis makes use of the fluorination of a pre-existing functional group using for example DAST or Deoxfluor [24] , [25] , [26] . Apart from the hazardous nature of these reagents, this approach is also limited with respect to functional group compatibility. In our opinion, the restricted availability of general and selective synthetic methodologies clearly impeded the development of versatile building blocks with functionalized difluoromethyl units. As an alternative strategy, the direct introduction of difluoroalkyl groups forming X−CF 2 –R bonds (X = C, O, N, S, etc. ; R = C) could solve this problem [27] , [28] , [29] , [30] , [31] , [32] , [33] . Especially, using gem -difluoroallyl moieties (a –CF 2 – group neighboring to an alkene unit) offers attractive possibilities because of the wide variety of subsequent functionalizations and its occurrence in existing pharmaceuticals (see also Fig. 1c ) [16] , [17] , [18] , [19] , [20] . Unfortunately, so far only a few methodologies for the direct intermolecular preparation of gem -difluoroallylic products are known [34] , [35] , [36] , [37] , [38] , [39] , [40] , [41] , [42] , [43] , [44] , [45] , [46] . This can be explained by the lack of suitable reagents like 3,3-difluoroallyl-X compounds [47] , [48] . Thus, 3-bromo-3,3-difluoropropene (BDFP) has become the most popular surrogate for such transformations [34] , [35] , [36] , [47] , which has been applied exemplarily to construct difluoroallylated alcohols via metal–halogen exchange reactions (Fig. 1d , left) [47] , [48] , [49] , [50] . In addition, Tsuji–Trost allylations of BDFP and related substrates were also disclosed (Fig. 1d , right) [34] , [35] , [36] , [37] , [38] . More specifically, the groups of Zhang [34] , Ichikawa [35] , and most recently Cogwell [36] , reported interesting Pd-catalyzed gem -difluoroallylation of organoboranes, halophenols, and anilines, respectively. Nevertheless, the use of BDFP has limitations due to its physical properties, e.g. volatility (b.p. : 41–42 °C) and substrate scope. In addition, the regioselective synthesis of the desired gem -difluoroallylated products requires the aid of stoichiometric amounts of metals or precious catalysts. In conclusion, to date, a general approach that meets the criteria of both broad reaction scope and high selectivity for gem -difluoroallylation reactions remains elusive. As a solution, herein we describe the development of a family of easily available and bench-stable gem -difluorinated allyl ammonium salts (DFAAs), which allow exclusive γ-regioselective gem -difluoroallylation of O -, N -, S -, Se -, and C -nucleophiles (Fig. 1e ). The resulting products, featuring a synthetically highly valuable Nu−CF 2 CH = CH 2 unit, allow for the straightforward synthesis of diverse organofluorine compound libraries that offer numerous possibilities to enlarge the chemical space in the development of bioactive molecules. Although quaternary allyl ammonium salts are known for more than a century [51] , they received surprisingly little attention [52] , [53] , [54] , [55] . While investigating palladium-catalyzed cascade processes for the synthesis of spiro-fused heterocycles [56] , recently we noticed the utility and advantages of this class of compounds compared to other allylic electrophiles such acetates, halides, and so on. Inspired by this work and our interest in organofluorine building blocks [56] , [57] , [58] , [59] , [60] , [61] , we became interested in the synthesis and applications of DFAAs. Surprisingly, the parent 3,3-difluoropropen-1-yl ammonium salts (DFPAs) have not been described before. Starting from 3,3,3-trifluoropropene, which is a commercial raw material, which is used for the preparation of a variety of products (e.g. in cosmetics, chemical manufacturing, etc. ), base-mediated amination with piperidine provided γ,γ-difluoroallyl piperidine smoothly as a colorless oil. Subsequent selective N -methylation [38] , gave the desired 3,3-difluoropropen-1-yl ammonium salt 1a as a crystalline white powder without the need for chromatography or other tedious purifications in 56% overall yield. Following this two-step protocol other γ,γ-fluoro-substituted derivatives 1b – 1e can be obtained on gram-scale in a straightforward manner (Fig. 2a ). Notably, all resulting products can be conveniently handled and are air-stable for months. Fig. 2: Reagent synthesis and model reaction. a Two-step synthesis procedure for the preparation of difluorinated allyl ammonium salts 1a – 1e . b Optimization studies for the S N 2′ substitution reaction of difluoroallyl ammonium salt 1a with 4-phenyl phenol 2 in the presence of different basic conditions. † PdBr 2 (0.015 mmol) and n BuPAd 2 (0.03 mmol) were used. ‡ The reaction was performed under an argon atmosphere. Full size image Having a small representative selection of fluorinated allyl ammonium salts in hand, we were interested to investigate their general reactivity. Here, we were especially interested in allylic substitution reactions with oxygen-derived or nitrogen-derived nucleophiles because the resulting structural motifs RCF 2 –O, RCF 2 –N are not easily accessible by other synthetic means. 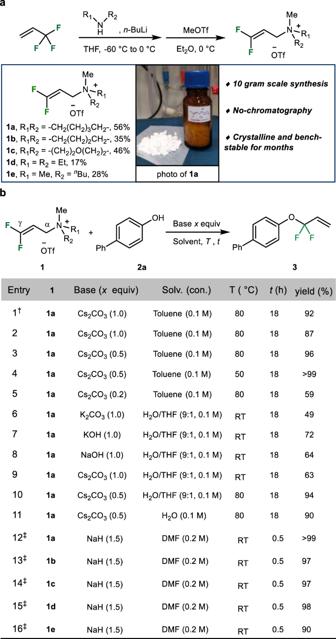Fig. 2: Reagent synthesis and model reaction. aTwo-step synthesis procedure for the preparation of difluorinated allyl ammonium salts1a–1e.bOptimization studies for the SN2′ substitution reaction of difluoroallyl ammonium salt1awith 4-phenyl phenol2in the presence of different basic conditions.†PdBr2(0.015 mmol) andnBuPAd2(0.03 mmol) were used.‡The reaction was performed under an argon atmosphere. Thus, the model reaction of γ,γ-difluoroallyl ammonium salt 1a with 4-phenyl phenol 2 was performed in the presence of a palladium catalyst under typical Tsuji–Trost conditions (toluene, 80 °C, PdBr 2 , n -butyl-diadamantylphosphine, cesium carbonate) [62] . To our delight, the desired difluoroallylic aryl ether product 3 is obtained in 92% yield and high selectivity (>99/1%; Fig. 2b , entry 1). Interestingly, performing a control experiment under identical conditions without the palladium catalyst revealed similar product yields (87% yield; Fig. 2b , entry 2), which can be explained by intrinsic reactivity for direct S N 2′ substitution in the presence of a base. Notably, even without any precious metal catalyst present, exclusive γ-selective substitution (>99/1) was observed without any detectable formation of the α-substitution product. In contrast, for other allylic electrophiles such behavior in the absence of transition metal catalysts is difficult to control [63] . Next, to obtain optimal results for this benchmark system, critical reaction parameters were studied in detail (see Supplementary Tables 1 – 3 ). The following observations are important to note: (a) It is possible to run the nucleophilic substitution efficiently under very mild conditions (RT to 50 °C) in the presence of sub-stoichiometric amounts of base without any metal catalyst (Fig. 2b , entries 3–10); (b) this transformation works well in aqueous solutions as well as pure water and high yields of 3 (up to 94%) can be obtained, which is interesting for biologically relevant substrates and considering the importance of green solvents (Fig. 2b , entries 6–11) [64] ; (c) using stronger base (sodium hydride), the reaction proceeded smoothly within minutes (typically <10 min) at ambient temperature affording the desired ether product 3 in quantitative yield (Fig. 2b , entry 12). Interestingly, depending on the physical properties of specific substrates, the most suited protocol might be selected from these orthogonal approaches. Similar results were obtained using other related ammonium salts 1b – 1e as difluoroallylating reagents (Fig. 2b , entries 13–16). After having demonstrated the efficiency of the model system at different conditions, we were interested in the general reaction scope. At first, other oxygen nucleophiles were studied. Using NaH as base, the gem -difluoroallylation of allylic ammonium salt 1a with various phenols provided allylic aryl ethers 3 – 18 in good to excellent yields. The reaction displayed remarkable compatibility with functional groups including ketones, aldehydes, esters, halides, amines, boronic acidic esters, heterocycles, and alkenes. As shown in the case of product 19 , the reaction can be easily run on gram-scale. Apart from phenols, a variety of aliphatic alcohols were successfully examined as well, affording the allylic alkyl ethers 23 – 27 in 63–99% yields. From a synthetic point of view, it is also interesting that gem -difluoroallylation of functionalized propargylic alcohols generated versatile diene-ynes ( 25 and 26 ) and 1,6-enyne ( 27 ). Notably, less common oxygen nucleophiles such as oximes and hydroxylamines also worked well and provided the respective products 20 – 22 in very good yields. Recently, these latter products attracted attention because of their potential application for fluoroalkoxylation of alkyl halides [65] . In addition to phenols, aliphatic and propargylic alcohols, also diverse sulfur-, selenium-, nitrogen-, as well as activated carbon-nucleophiles can be used according to our general protocol as depicted in Fig. 3 . More specifically, aryl thiols bearing electron-donating or electron-withdrawing groups and alkyl thiols as well as benzeneselenol underwent the desired the S - or Se - gem -difluoroallylation leading to the corresponding products 28 – 32 . Gratifyingly, these reaction conditions can be used for a broad range of heterocyclic amines and tosyl-protected secondary amines, too. In all cases, the reaction proceeded smoothly to give 33 – 38 bearing allylic N -difluoromethylene unit in high yields. Fig. 3: Regioselective substitution of 1a by different O-, N-, S-, Se- and C-nucleophiles: Substrate scope. Standard reaction conditions: 1 (1.2 equiv), 2 (1 equiv), NaH (1.5 equiv) in DMF (0.2 M), the reaction mixture was performed at 23 °C under argon atmosphere for 30 min, isolated yield, the α/γ regioselectivity was determined by crude 19 F NMR analyses. † Cs 2 CO 3 (0.5 equiv) and toluene (0.1 M) were used as base and solvent, the reaction was performed at 50 °C under air atmosphere for 18 h. Full size image Next, we turned our attention to the reaction of activated carbon nucleophiles. Interestingly, using ketones with β-H resulted selectively in O - gem -difluoroallylation and provided the corresponding allyl vinyl ethers 39 – 42 as single products in 73–99% yields. The high carbon/oxygen (C/O) regioselectivity could be explained by the Pearson acid–base concept [66] , [67] . On the other hand, using diphenylacetonitrile led to the construction of C sp3 –CF 2 R bond ( 43 ) and thus to access α-difluoroalkylated carboxylic acid derivatives. It is important mentioning that in all cases, the α/γ-regioselective gem -difluoroallylation undoubtedly generated exclusively the γ-substitution product. At this point it should be also noted that many difluoroallyl ammonium salts can be used for the preparation of more substituted derivatives following a similar methodology (see Supplementary Fig. 3). To showcase the value of this synthetic approach, late-stage functionalization of a variety of pharmaceuticals, bioactive molecules, and natural products are depicted in Fig. 4 . More specifically, estrone, one of the three major endogenous estrogens, with a phenolic group delivered to the difluoroallylic derivative 44 in excellent yield (97%). The molecular structure of 44 was confirmed by X-ray crystallography. Similar transformations performed with the (+)-α-tocopherol, acetate-protected β -estradiol, and diethylstilbestrol afforded the desired products 45 – 47 with high efficiency (99%, 97%, and 92%, respectively). Furthermore, monoterpene ( Z )-nerol—known as sweet rose-like aroma—bearing an allylic hydroxyl group, gave the corresponding 1,6,10-triene 48 in 97% yield. Additionally, several functionalized biologically relevant primary and secondary alcohols and various pharmaceutically important molecules, such as mestranol, lynestrenol, quinine, and testosterone, containing sterically congested tertiary or secondary hydroxyl groups, underwent this reaction smoothly, giving 49 – 55 in good to excellent yields. Notably, a derivative of the sulfonamide Celecoxib (analgesic) also could be coupled to give the N -difluoroallylated product 56 in high yields. 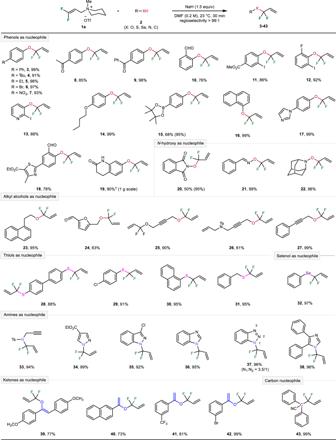Fig. 3: Regioselective substitution of 1a by different O-, N-, S-, Se- and C-nucleophiles: Substrate scope. Standard reaction conditions:1(1.2 equiv),2(1 equiv), NaH (1.5 equiv) in DMF (0.2 M), the reaction mixture was performed at 23 °C under argon atmosphere for 30 min, isolated yield, the α/γ regioselectivity was determined by crude19F NMR analyses.†Cs2CO3(0.5 equiv) and toluene (0.1 M) were used as base and solvent, the reaction was performed at 50 °C under air atmosphere for 18 h. Fig. 4: Selective 1,1-difluoroallylation of natural products and pharmaceuticals. Standard reaction conditions: 1a (1.2 equiv), 2 (1 equiv), NaH (1.5 equiv) in DMF (0.2 M), the reaction mixture was performed at 23 °C under argon atmosphere for 30 min, isolated yield, the α/γ regioselectivity was determined by crude 19 F NMR analyses. † Cs 2 CO 3 (0.5 equiv) and toluene (0.1 M) were used as base and solvent, the reaction was performed at 50 °C under air atmosphere for 18 h. Full size image Difluoroallylic S N 2′ substitution of different substrates containing more than one activated proton further highlights the importance of this method, especially in the late-stage functionalization of bioactive molecules. To ensure chemoselectivity, the milder base Cs 2 CO 3 was applied in these examples. For example, ezetimibe, an FDA-approved drug for the treatment of high blood cholesterol and certain other lipid abnormalities, underwent selective gem -difluoroallylation to give 60 in 84% yield. This demonstrates the compatibility of the reaction conditions with aliphatic hydroxyl groups and an amide-activated β-protons. In addition, transformations of N -Boc-protected L -tyrosine derivative, ethynylestradiol, and β-estradiol afforded the desired products 57 – 59 in high yields. After validating the generality of our protocol and having a selection of allylic gem -difluoride building blocks in hand, we wanted to demonstrate their value by further valorizations (Fig. 5 ). Exemplarily, we first carried out the Pd-catalyzed alkoxycarbonylation of gem -difluoroallylic aryl ether 3 without further optimizations. Taking advantage of the specific phosphine ligand L1 with built-in-base functions [68] , [69] , the corresponding product 61 was obtained in 73% yield with high regioselectivity for the linear product. Furthermore, under-reported reaction conditions [70] , 3 underwent highly regioselective hydroformylation using simple Co 2 (CO) 8 as the pre-catalyst (87% yield, l / b > 20/1). Fig. 5: Synthesis of gem -difluorinated analogs of drugs and further valorization of gem -difluorinated allyl ethers. a Transition-metal catalyzed carbonylation of difluorinated alkene 3 . b Dihydroxylation of 16 and 23 to give difluorinated 1-aryl-glycerols. c Ruthenium-catalyzed [2 + 2 + 2] co-cyclization of diene-yne 26 . d Rhodium-catalyzed reductive cyclization of 1,6-enyne 25 . e Practical procedures for the synthesis of OCF 2 -Aripiprazole 70 . f Four-step protocol for the synthesis of OCF 2 - Pramocaine 73 . 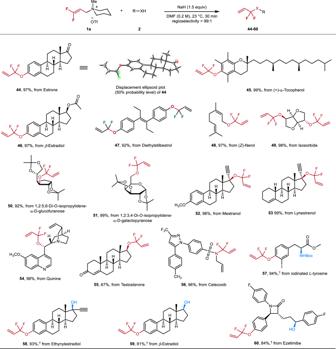Fig. 4: Selective 1,1-difluoroallylation of natural products and pharmaceuticals. Standard reaction conditions:1a(1.2 equiv),2(1 equiv), NaH (1.5 equiv) in DMF (0.2 M), the reaction mixture was performed at 23 °C under argon atmosphere for 30 min, isolated yield, the α/γ regioselectivity was determined by crude19F NMR analyses.†Cs2CO3(0.5 equiv) and toluene (0.1 M) were used as base and solvent, the reaction was performed at 50 °C under air atmosphere for 18 h. 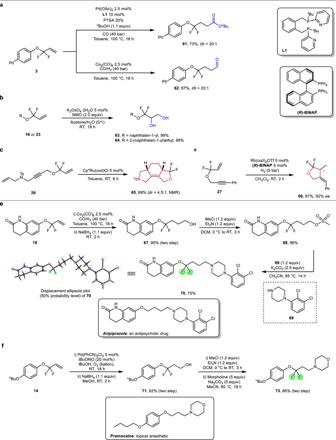Fig. 5: Synthesis ofgem-difluorinated analogs of drugs and further valorization ofgem-difluorinated allyl ethers. aTransition-metal catalyzed carbonylation of difluorinated alkene3.bDihydroxylation of16and23to give difluorinated 1-aryl-glycerols.cRuthenium-catalyzed [2 + 2 + 2] co-cyclization of diene-yne26.dRhodium-catalyzed reductive cyclization of 1,6-enyne25.ePractical procedures for the synthesis ofOCF2-Aripiprazole70.fFour-step protocol for the synthesis ofOCF2-Pramocaine73. Full size image Apart from aldehydes and carboxylic acids, the difluorinated products constitute virtuous precursors for the synthesis of other multifunctional compounds. For example, dihydroxylation of 16 and 23 provided the corresponding difluoromethylated glycerol derivatives 63 and 64 in quantitative yields (Fig. 5b ). These compounds are of interest as potential precursors for the preparation of difluorinated propranolol and many other analogs of beta blocker pharmaceuticals [71] . Considering transition-metal-catalyzed carbocycloaddition reactions as powerful methods for the construction of poly-heterocycles [72] , products 26 and 27 were examined following previously reported protocols. Indeed, starting from diene-yne 26 , an intramolecular ruthenium-catalyzed [2 + 2 + 2] co-cyclization took place to yield the N , O -fused tricyclic heterocycle 65 in 69% yield, albeit with moderate diastereoselectivity. The asymmetric version of rhodium-catalyzed reductive cyclization of 1,6-enyne 27 successfully proceeded at ambient temperature and hydrogen pressure, affording the gem -difluorinated alkylidene-substituted furan 66 in excellent yield and high enantioselectivity (97% yield, 92% ee ). Finally, two gem -difluoromethylene-containing analogs of actual drug compounds were prepared using the here presented methodology. Aripiprazole is an antipsychotic drug, ranking 128th among the top 200 retail drugs in 2019 with annual sales >1.2 billion dollars [73] . In a straightforward manner the O–CF 2 -derivative of aripirazole was successfully synthesized from commercially available materials, as illustrated in Fig. 5e . After highly regioselective hydroformylation of difluoroallylic aryl ether 19 , followed by subsequent reduction, mesylation, and final S N 2 substitution, the desired difluorinated aripiprazole 70 was obtained in 68% overall yield. As the second example, the CF 2 -analog of Pramocaine (a topical anesthetic) was prepared easily in four steps in 53% overall yield (Fig. 5f ). In summary, we present the parent examples of DFPAs, which can be easily prepared by base-mediated amination of the industrial feedstock 3,3,3-trifluoropropene. The resulting compounds are air-stable and water-stable and can be conveniently applied as highly efficient difluoromethylene reagents. Following an operationally simple and scalable protocol various nucleophiles including phenols, alcohols, thiols, selenols, amines, ketones, and alkanes with activated C sp3 -H undergo exclusively γ-regioselectivity gem -difluoroallylation without the need of transition-metals under mild conditions. So far, the resulting allylic gem -difluoromethylated products were difficult to access by using conventional approaches. The successful incorporation of the allylic difluoromethylene unit into a wide variety of bioactive pharmaceuticals and natural products provides chemists a new route to explore fluorine-containing molecular scaffolds. General procedure A for the preparation of allylic gem-difluoromethylated compounds To a 25 mL oven-dried pressure tube equipped with a magnetic stir bar were added difluoroallyl ammonium salt 1 (0.36 mmol), NaH (0.45 mmol), DMF (1.5 mL), and then nucleophiles 2 (0.3 mmol) was introduced under argon atmosphere. The sealed pressure tube was vigorously stirred at 23 °C for 30 min. The reaction mixture was quenched with few drops of water and extracted with ethyl acetate (3 × 20 mL). The combined organic layer was dried over anhydrous Na 2 SO 4 , filtered and concentrated. The residue was purified by chromatography on silica gel (It is worthy to note that some of the fluorinated product can only be separated without decomposition with 2% triethylamine in the eluent) to afford the desired product. General procedure B for the preparation of allylic gem-difluoromethylated compounds To a pressure tube (25 mL) equipped with a magnetic stir bar difluoroallyl ammonium salt 1 (0.36 mmol), Cs 2 CO 3 (0.15 mmol), toluene (2.5 mL), and then nucleophiles 2 (0.3 mmol) were added. The sealed pressure tube was vigorously stirred for 18 h at 50 °C under air atmosphere. After cooling to r.t., the reaction mixture was diluted with ethyl acetate (10 mL) and filtered through a short pad of celite eluting with ethyl acetate (3 × 10 mL). After evaporation, the residue was purified by chromatography on silica gel to afford the desired product. Notably, some of the fluorinated products can only be separated without decomposition with 2% triethylamine in the eluent.